Microfluidic quadrupole and floating concentration gradient The concept of fluidic multipoles, in analogy to electrostatics, has long been known as a particular class of solutions of the Navier-Stokes equation in potential flows; however, experimental observations of fluidic multipoles and of their characteristics have not been reported yet. Here we present a two-dimensional microfluidic quadrupole and a theoretical analysis consistent with the experimental observations. The microfluidic quadrupole was formed by simultaneously injecting and aspirating fluids from two pairs of opposing apertures in a narrow gap formed between a microfluidic probe and a substrate. A stagnation point was formed at the centre of the microfluidic quadrupole, and its position could be rapidly adjusted hydrodynamically. Following the injection of a solute through one of the poles, a stationary, tunable, and movable—that is, 'floating'—concentration gradient was formed at the stagnation point. Our results lay the foundation for future combined experimental and theoretical exploration of microfluidic planar multipoles including convective–diffusive phenomena. Quadrupoles are used in numerous physical and engineering applications and arise under many forms, such as electrical charges and currents [1] , magnetic poles [2] , acoustic poles [3] , [4] , and gravitational masses [5] . Two popular applications of quadrupoles include the quadrupole mass spectrometer that uses four parallel metal rods with opposing alternating electrical currents to filter ions based on their mass-to-charge ratio [6] , and the quadrupole magnets that are used to focus beams of charged particles in particle accelerators [2] . In fluid mechanics, flow dipoles, or 'doublets' have been studied in porous rocks notably in the context of oil extraction [7] , [8] . To increase the recovery of oil pumped from a well, a solution can be injected in another well to displace the oil trapped within the rocks, according to a dipolar flow profile. We recently introduced the microfluidic probe (MFP) [9] that uses both injection and aspiration aperture to flush a stream across a substrate surface, and that in fact represents a two-dimensional fluidic dipole, although this analogy has not been developed. Planar multipoles with more than two flow poles have been investigated theoretically by Koplik et al . with increasing numbers of sources and sinks (such as quadrupoles, octopoles etc.) [10] . Bazant et al . have also demonstrated the use of conformal mapping to solve a broad class of advection–diffusion problems in 2D irrotational flows [11] by drawing an analogy with the pioneering work of Burgers on out-of-plane flow velocity in 2D vortex sheets [12] . However, experimental validation of these theoretical analyses is still outstanding as flow multipoles have not, to the best of our knowledge, been produced experimentally. In this work, we present an experimental planar microfluidic quadrupole (MQ) in an open space confined between two parallel plates ( Fig. 1 ). We extend the theoretical framework to describe hydrodynamic and convective–diffusive properties of the MQ in Hele–Shaw flows and derive the equations for the key parameters characteristic of the MQ such as the size of the flow confinement and length of the gradient formed within the MQ. Finite element simulations complete the analytical results and both are compared with experimental results. Finally, we present a first application of the MQ that can be used as a gradient generator and which, unlike prior gradient generators, affords low shear stress, rapid spatiotemporal tuning of the gradient either hydrodynamically by adjusting the flow rates, or physically by moving the MFP, and can be applied on any planar substrate and displaced as well. 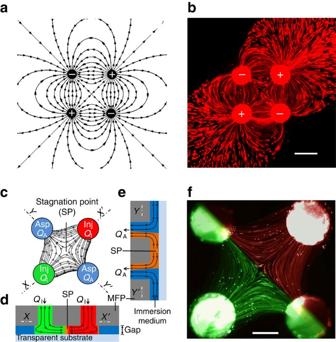Figure 1: Two-dimensional MQ formed in gap between a MFP and a substrate. (a) Schematics of the field lines in a 2D electrostatic quadrupole consisting of two pairs of opposing positive and negative charges. (b) Experimental image of a MQ when formed by injecting and aspirating liquids with tracer beads via two injections (plus sign) and two aspirations (minus sign) apertures. Path lines were captured by the long-term exposure of the flowing fluorescent tracer beads. Whereas we adopt the same symbolism than for electrical charges, the '+' and '−' signs correspond to purely fluidic sources and sinks. Scale bar is 400 μm. (c) Schematic of a MQ generated between two parallel plates formed by a MFP with four apertures on top and a transparent substrate at the bottom. The flow lines between the apertures represent a scenario where the aspiration flow rates are larger than the injection flow rates and thus all the injected liquid is confined and re-aspirated. A SP is formed at the centre. (d) X–X′ and (e) Y–Y′ cross-sectional views of the MQ under the MFP (not to scale). (f) Fluorescence micrograph showing path lines in a MQ using 2 μm red and green tracer microbeads injected (Qinj=10 nl s−1) through the top right and bottom left apertures, respectively, into a 50 μm gap filled with liquid, and aspirated back (Qasp=100 nl s−1) through the other two apertures. Scale bar is 200 μm. Figure 1: Two-dimensional MQ formed in gap between a MFP and a substrate. ( a ) Schematics of the field lines in a 2D electrostatic quadrupole consisting of two pairs of opposing positive and negative charges. ( b ) Experimental image of a MQ when formed by injecting and aspirating liquids with tracer beads via two injections (plus sign) and two aspirations (minus sign) apertures. Path lines were captured by the long-term exposure of the flowing fluorescent tracer beads. Whereas we adopt the same symbolism than for electrical charges, the '+' and '−' signs correspond to purely fluidic sources and sinks. Scale bar is 400 μm. ( c ) Schematic of a MQ generated between two parallel plates formed by a MFP with four apertures on top and a transparent substrate at the bottom. The flow lines between the apertures represent a scenario where the aspiration flow rates are larger than the injection flow rates and thus all the injected liquid is confined and re-aspirated. A SP is formed at the centre. ( d ) X–X′ and ( e ) Y–Y′ cross-sectional views of the MQ under the MFP (not to scale). ( f ) Fluorescence micrograph showing path lines in a MQ using 2 μm red and green tracer microbeads injected ( Q inj =10 nl s −1 ) through the top right and bottom left apertures, respectively, into a 50 μm gap filled with liquid, and aspirated back ( Q asp =100 nl s −1 ) through the other two apertures. Scale bar is 200 μm. Full size image Microfluidic quadrupole MQs were formed between a MFP [9] with 4 apertures arranged in a classical symmetric quadrupole configuration ( Fig. 1b ) and a flat bottom substrate. The MFP was microfabricated into Si and diced into squares with four openings constituting pairs of opposing apertures used for injection and aspiration. A Polydimethylsiloxane (PDMS) adapter block was bonded to the die, and capillaries were plugged into the block and connected to syringe pumps ( Fig. 2a,b ). 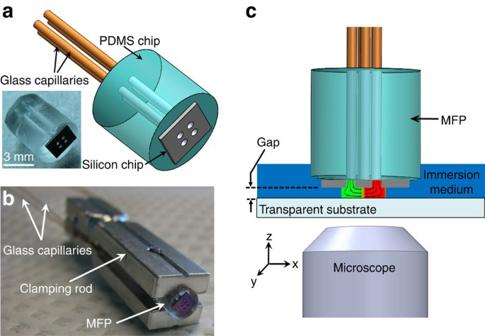Figure 2: Experimental MFP apparatus. (a) A 3D illustration of the MFP along with a micrograph shown in the inset. (b) A MFP connected to the syringe pumps using capillaries and fixed within the clamping rod and mounted on a XYZ micropositioner that together form the MFP holder. (c) Using the MFP holder (not shown), the MFP is aligned parallel to the substrate and positioned above it with micrometer accuracy thus forming a microscopic gap. The MFP is immersed in a liquid that thus fills the gap. The bottom substrate, usually a glass slide or a cover slip, is placed on the motorized stage of a microscope (not shown) and can be moved with respect to the MFP (and the objective) using a joystick or controlled using a computer program. Schematics are not to scale. Figure 2: Experimental MFP apparatus. ( a ) A 3D illustration of the MFP along with a micrograph shown in the inset. ( b ) A MFP connected to the syringe pumps using capillaries and fixed within the clamping rod and mounted on a XYZ micropositioner that together form the MFP holder. ( c ) Using the MFP holder (not shown), the MFP is aligned parallel to the substrate and positioned above it with micrometer accuracy thus forming a microscopic gap. The MFP is immersed in a liquid that thus fills the gap. The bottom substrate, usually a glass slide or a cover slip, is placed on the motorized stage of a microscope (not shown) and can be moved with respect to the MFP (and the objective) using a joystick or controlled using a computer program. Schematics are not to scale. Full size image The MFP was immersed in fluid and brought close to a planar substrate so as to form a narrow gap (see Methods). A glass slide was used as the bottom substrate permitting visualization of the flow within the gap using an inverted microscope ( Fig. 2c ). Simultaneous injection and aspiration of fluid generates the quadrupolar flow, and the two injected fluids meet head-on at the centre of the MQ, generating a stagnation point (SP) with zero flow velocity ( Fig. 1c–f ). When the aspiration and injection flow rates are identical, a large fraction of the injected stream is re-aspirated; but the fraction of fluid that radially flows outward is not ( Fig. 1b ) and thus leaks into the fluid surrounding the MFP. However, if the ratio of aspiration/injection flow rates is >1, all the injected liquid is captured and aspirated back into the MFP ( Fig. 1f ). We arbitrarily define the two injection apertures as positive poles (sources) and the aspiration apertures as negative poles (drains) ( Supplementary Figure S1 ; Supplementary Methods ). The MFP used here featured a centre-to-centre separation of 1,075 μm between pairs of opposing apertures, each 360 μm in diameter, and was positioned above, parallel to the bottom substrate so as to form a 50 μm gap for all experiments. This setup represents a parallel-plates configuration, and the MQ formed in the gap is quasi-two-dimensional. Using the Hele–Shaw approximation, it can thus be conveniently described as a two-dimensional Stokes flow of the form [13] : where is the velocity field of the MQ, η is the viscosity, p is the hydrostatic pressure, H is the height of the gap between the plates ( H =50 μm), and z is the vertical coordinate whereas z =0 corresponds to the bottom plate (substrate) and z = H to the top plate (MFP). The resulting flow velocities in the MQ are on the order of 2 mm s −1 or less for aspiration flow rates of 100 nl s −1 and the flow is purely viscous (Re ≪ 1), Supplementary Methods for details. Averaging equation (1) over the gap height, the velocity profile can be simplified as: The height-averaged velocity profile given by this expression is irrotational [13] , and can therefore be represented by a scalar potential akin to an electric field or a current distribution that can also be described based on an electrostatic potential ( Table 1 ). It thus becomes possible to calculate the flow velocity for any coordinate of the MQ by using the superposition principle as in the case of electrical charges and current quadrupoles (see Supplementary Methods ): where is the position vector and is the position of the sources and drains, both with respect to the centre of the probe. Q i is the flow rate from the i th inlet corresponding to Q inj and Q asp for injected and aspirated flow rate, respectively. Table 1 Fundamental equations and equivalences for electrical charge (electrostatics), electrical current (electrokinetics), and fluid velocity (fluid mechanics) under the Hele–Shaw approximation. Full size table Flow confinements of the MQ As mentioned earlier, the flow rates ratio Q asp / Q inj needs to be sufficiently high to hydrodynamically confine and capture all the injected fluid ( Fig. 1b versus Fig. 1f ). The confinement of the injected streams as function of the flow rates ratio were visualized using fluorescent tracer particles ( Fig. 3a–c ). The area flushed by the injected streams is an important concept for fluidic applications, because chemicals injected in the streams may be used to process selectively the underlying surface [9] , and we thus establish an analytical solution. The fluid that radiates outwards, relative to the centre of the MQ, will travel the greatest distance until the flow velocity becomes zero, at which point the flow direction is reversed, and it is eventually recaptured by an aspiration aperture. The confinement radius R of the MQ was defined as the distance between the SP and the outermost point of zero velocity for the radial streams, and using equation (3) yields ( Supplementary Methods ): where Q asp is the aspiration flow rate, Q inj is the injection flow rate, and d is the centre-to-centre distance between the two inlets. We found excellent agreement between the calculated and experimentally measured R ( Fig. 3 ). These results confirm the validity of our theoretical assumptions and analysis. 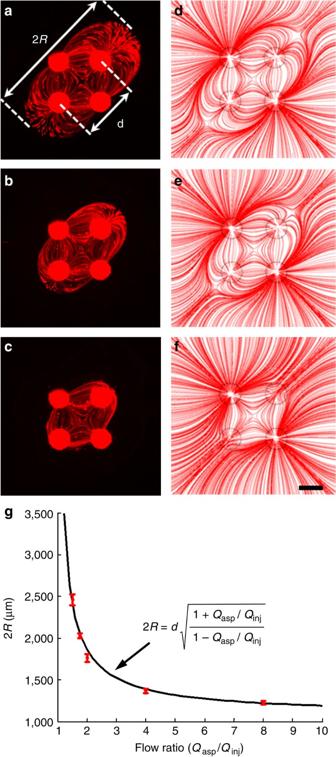Figure 3: Flow confinement in a MQ for varying ratio of aspiration to injection flow rates. 2 μm fluorescent tracer microbeads were injected at 50 nl s−1through the top right and bottom left apertures (+) and aspirated back through the other two apertures (−). For all experimental data, fluorescent paths of microbeads revealing the streamlines were captured with a 1 s exposure. (a–c) Flow pattern for a ratioQasp/Qinj=1.75, 2, and 4, respectively. (d–f) Streamlines obtained by FEM simulations for the flow ratios used in (a–c), respectively. (g) Comparison of theoretical and experimental (shown as red dots) 2Ras a function of the flow ratio reveals a good agreement. Error bars represent the standard error of four separate experiments. Scale bar is 400 μm. Figure 3: Flow confinement in a MQ for varying ratio of aspiration to injection flow rates. 2 μm fluorescent tracer microbeads were injected at 50 nl s −1 through the top right and bottom left apertures (+) and aspirated back through the other two apertures (−). For all experimental data, fluorescent paths of microbeads revealing the streamlines were captured with a 1 s exposure. ( a – c ) Flow pattern for a ratio Q asp / Q inj =1.75, 2, and 4, respectively. ( d – f ) Streamlines obtained by FEM simulations for the flow ratios used in ( a – c ), respectively. ( g ) Comparison of theoretical and experimental (shown as red dots) 2 R as a function of the flow ratio reveals a good agreement. Error bars represent the standard error of four separate experiments. Scale bar is 400 μm. Full size image Fluid flow around the SP A two-variable ( x , y ) Taylor expansion of equation (3) yields the velocity profile in the very close vicinity of the SP (valid for x ,y ≪ d), see Supplementary Methods for details: where 〈 Q 〉=( Q asp + Q inj )/2 is the average flow rate between the inlet and outlet, and the origin (0,0) corresponds to the position of the SP. The flow profile can also be expressed in the form of a velocity potential [11] , ( Table 1) : Interestingly, this velocity potential is identical to the one describing two-dimensional flow along a right-angle corner [14] . In the MQ, the four quadrants defined by the symmetry lines XX ′ and YY ′ in Figure 1d each constitute a virtual corner with a corresponding corner flow. Path lines formed by green tracer beads and a ratio Q asp / Q inj =10 outline the SP at the centre ( Fig. 1f ; Supplementary Movie 1 ), and are consistent with the velocity profile and streamlines obtained using FEM simulations ( Fig. 4a ). As the flow velocity tends to zero when approaching the SP ( Fig. 4b ), the calculated wall shear stress was found to converge to zero as well, Supplementary Figure S2a . The shear stress increases linearly when moving away from the SP and reaches a maxima near the inner edge of each aspiration aperture. 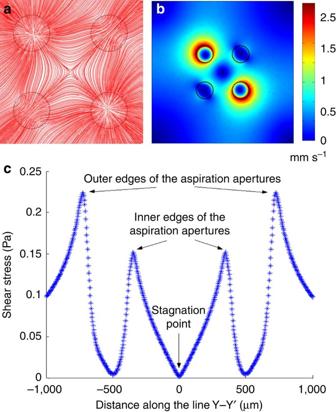Figure 4: Fluid flow and shear stress in the MQ. FEM simulation of the MQ with 100 and 10 nl s−1aspiration and injection flow rates, respectively. (a) Streamlines revealing the SP at the centre. (b) Flow velocity profile at the mid-plane (z=25 μm) in the MQ revealing the zero fluid flow at the SP and the low flow in the areas surrounding the SP as well as at the centre of the poles. (c) Total shear stress profile at the substrate along a line connecting the two aspiration apertures and crossing the SP (lineY–Y′ shown inSupplementary Fig. S2a). The shear stress between the four apertures increases almost linearly from zero at the SP to a first maxima at the inner edge of each aspiration aperture (τ=0.15 Pa), drops back to almost zero at the centre, and reaches the maxima at the outer edge of the aperture. Within a circle with a diameter of 100 μm ( ∼ 10% of the distance d ) centred at the SP, shear stresses are less than 10% of that local maxima as shown in Figure 4c ( Supplementary Methods ). For a MQ with injection and aspiration flow rates of 10 and 100 nl s −1 , respectively, the local maxima of shear stresses is τ max =0.15 Pa, and hence <0.015 Pa inside the circle. The shear stress also varies linearly with the aspiration flow rates that may be reduced to further minimize stress ( Supplementary Fig. S2b ; Supplementary Methods ). Figure 4: Fluid flow and shear stress in the MQ. FEM simulation of the MQ with 100 and 10 nl s −1 aspiration and injection flow rates, respectively. ( a ) Streamlines revealing the SP at the centre. ( b ) Flow velocity profile at the mid-plane ( z =25 μm) in the MQ revealing the zero fluid flow at the SP and the low flow in the areas surrounding the SP as well as at the centre of the poles. ( c ) Total shear stress profile at the substrate along a line connecting the two aspiration apertures and crossing the SP (line Y – Y ′ shown in Supplementary Fig. S2a ). The shear stress between the four apertures increases almost linearly from zero at the SP to a first maxima at the inner edge of each aspiration aperture ( τ =0.15 Pa), drops back to almost zero at the centre, and reaches the maxima at the outer edge of the aperture. Full size image Convection–diffusion and gradients at the SP When a solute is added to one of the injected streams, diffusive mass transport gradually dominates when approaching the SP as the convective flow converges towards zero. The solute is continuously replenished by one stream acting as a source, while it is also continuously transported away by the other stream that acts as a sink. Along the axis of the two injection apertures ( XX ′), the solute diffuses into the opposing stream at the SP while it is simultaneously pushed back by the inward convection of the opposing stream, and a steady-state, stationary concentration gradient is formed. To characterize this gradient mathematically, we first consider the general time-dependent diffusion–convection equation [15] : where D is the diffusivity of the species studied, is the height-averaged in plane velocity profile and C is the concentration of the solute (normalized between 0 and 1). The steady-state version of equation (7) (with the left-hand term set to zero) is reminiscent of the flow in a 'Burgers vortex sheet' [12] where C is analogous to the out of plane velocity, as was pointed out by Bazant and Moffatt [16] . On the basis of the experimental observations shown below, the gradient length, which here is defined as the distance between the points with a concentration of 10 and 90% of the original solute concentration, is small when compared with the distance between the inlets along the XX ′ axis ( Fig. 5a ). Using the approximated velocity profile around the SP of equation (5), and combining it with equation (7), the convection–diffusion equation relevant to the flow around the SP formed within the MQ can be re-written as: where D is the diffusion constant of the solute. The derivatives with respect to y have been neglected in equations (7) and (8) as the concentration interface is invariant in y ( ∂C / ∂y =0 everywhere) under Hele–Shaw assumption; see Supplementary Methods for details. 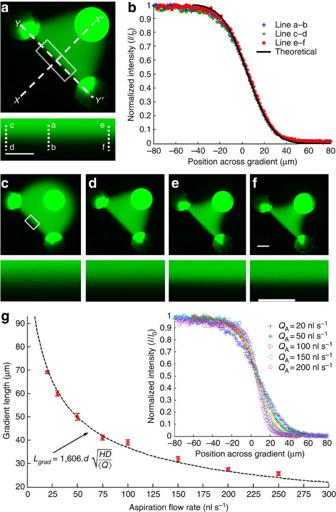Figure 5: Tunable concentration gradients formed at the SP of a MQ. (a) 50 and 10 nl s−1were used as aspiration (Qasp) and injection (Qinj) flow rates, respectively, and fluorescein was added to the solution injected through the top right aperture. A close-up view of the gradient corresponding to the white rectangle is shown as inset. (b) Fluorescence intensity profiles of the gradients across the linesa–b,c–d, ande–fin (a) show good agreement between theory and experiment and that the gradient shape does not change along the Y–Y′ axis. (c–f) Images of the fluorescein distribution and concentration gradients within the MQ for an injection flow rateQinj=10 nl/s and for a flow rate ratioQasp/Qinj=2, 10, 15, and 20, respectively (insets are close-up views). Scale bar is 200 μm in the overviews and 100 μm in the close-up views. (g) The measured length of the gradient with different aspiration flow rates are shown as red dots. Error bars represent the standard error of five separate experiments. The analytical solution is shown as a dashed line and shows excellent agreement with the experiment. Fluorescence intensity profiles along the central line across each gradient for different aspiration flow rates are shown in the inset. Using the dimensionless numbers , , where is the global Péclet number for the MQ, we find the simple dimensionless expression for this transport problem to be: Figure 5: Tunable concentration gradients formed at the SP of a MQ. ( a ) 50 and 10 nl s −1 were used as aspiration ( Q asp ) and injection ( Q inj ) flow rates, respectively, and fluorescein was added to the solution injected through the top right aperture. A close-up view of the gradient corresponding to the white rectangle is shown as inset. ( b ) Fluorescence intensity profiles of the gradients across the lines a – b , c – d , and e – f in ( a ) show good agreement between theory and experiment and that the gradient shape does not change along the Y–Y′ axis. ( c – f ) Images of the fluorescein distribution and concentration gradients within the MQ for an injection flow rate Q inj =10 nl/s and for a flow rate ratio Q asp / Q inj =2, 10, 15, and 20, respectively (insets are close-up views). Scale bar is 200 μm in the overviews and 100 μm in the close-up views. ( g ) The measured length of the gradient with different aspiration flow rates are shown as red dots. Error bars represent the standard error of five separate experiments. The analytical solution is shown as a dashed line and shows excellent agreement with the experiment. Fluorescence intensity profiles along the central line across each gradient for different aspiration flow rates are shown in the inset. Full size image Therefore and are the natural scales of the MQ. They represent, respectively, the length over which diffusion takes place at the interface and the characteristic time before steady state is achieved. Typical conditions in our experiments were an average flow rate of 55 nl s −1 , and D =500 μm 2 s −1 as we used fluorescein as the diffusive species. Using these values, we obtain x 0 =15 μm and t 0 =0.4 s. Thus, after a few seconds, the gradient will have reached a steady –state, and the time-dependent term of equation (9) can be neglected. When performing this approximation, equation (9) reduces to a one-dimensional problem with C ( x , t ) being the concentration profile at the SP perpendicularly to the interface where diffusion takes place. For the experimental conditions used here, the concentration gradients at the SP were much shorter than the distance d separating the two inlets, d may thus be considered infinite and thus the boundary conditions become: This allows simplifying the calculations and solving equations (9) and (10) for the concentration under these conditions gives: where erf is the error function [17] . Once again, the solution here is similar to that of the out-of-plane velocity in a Burgers vortex sheet, but with the Péclet number replacing the Reynolds number of the classical analysis [16] . The gradient length can be calculated using equation (11) and expressed as: The gradient length is proportional to the average flow rate and obeys a simple power law. The analytical solution for the gradient length was compared with experimental measurements using fluorescein sodium salts (376 Da, diffusion coefficient in water D =500 μm 2 s −1 (refs 18 , 19 , 20 )) diluted in water. Fluorescein was injected through the top-right aperture, and the gradient formation at the SP within the MQ was modelled numerically ( Supplementary Fig. S3a ), and measured experimentally, ( Fig. 5a ). Theoretical and experiment gradient profiles are in excellent agreement, ( Fig. 5b ; Supplementary Figure S3b ). We observed that the gradient was constant along the YY ′ axis connecting the two aspiration apertures( Fig. 5a,b ). The flow perpendicular to the gradient carries it towards each of the aspiration apertures, and convection rapidly dominates diffusion when moving away from the SP (see Supplementary Methods for details) while the concentric flow around the aspiration apertures focuses the stream when approaching the inlet. Collectively, these effects counter diffusive broadening of the gradient and explain the quasi-constant gradient profile along the YY ′ line connecting both aspiration apertures. We compared the calculated gradient length with experimental measurements for a Q asp / Q inj, varying from 2 to 15 ( Fig. 5c–g ), and found them to be in good agreement. For Q asp increasing from 20 to 250 nl s −1 , the gradient length decreased from 69 to 25.7 μm. This range of accessible gradient slopes may be further increased by exploring a wider range of flow rates from pl s −1 to μl s −1 . The gradient changes rapidly ( Supplementary Movie 2 ), and, therefore, dynamic gradients may readily be formed simply by pre-programming the aspiration flow rates. Whereas the confinement of the MQ is governed by Q asp / Q inj , equation (12) indicates that the gradient slope and length depend on 〈 Q 〉 and, thus, primarily on Q asp for high ratios of Q asp / Q inj . This theoretical result is supported by the experiments where only Q asp was changed, Figure 5 , or where only Q inj was tuned ( Supplementary Figure S4 ; Supplementary Movie 3 ). It is thus possible to vary the confinement and the gradient slope independently by keeping one of them constant by simultaneously tuning Q asp and Q inj . Asymmetric MQ flow profiles and floating gradient For all experiments described up to this point, each pair of injection and of aspiration flow rates were adjusted in synchrony and kept equal, which fixed the SP at the centre of the MQ. If the flow rate of only one of the two injection or aspiration apertures is changed, the symmetry is broken and the position of the SP will change ( Fig. 6a,b ). The gradient, which originates at the SP, moves along with the SP and can thus be displaced hydrodynamically within the central area of the MQ. The gradient is formed along a straight interface when the SP is centred, and along a curved interface when moving the SP towards any of the injection apertures ( Fig. 6c,d ). By using a programmable flow control system, or by manually changing the flow rates, oscillating and rapidly moving gradients can be generated ( Supplementary Movie 4 ). Complex spatiotemporal gradient landscapes may thus be formed around a particular point by changing both the gradient slope and the gradient position. The gradient may be adjusted either in a preprogrammed manner, or in real time in response to observations. 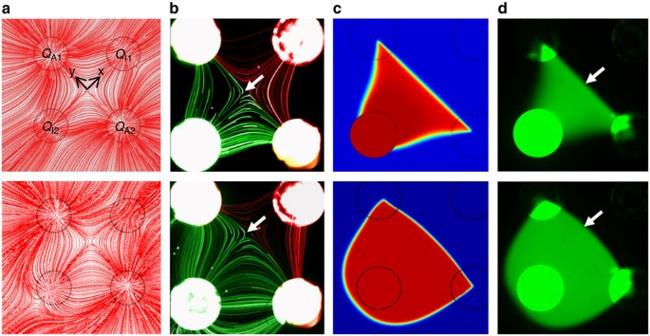Figure 6: Hydrodynamic positioning of the SP. The SP and the gradient floating between the streams were tuned by independently adjusting the flow rate of each pole of the MQ. (a) Streamlines of the flow showing the SP at the centre (upper) of the MQ forQI1=QI2=10 nl s−1andQA1=QA2=100 nl s−1, and shifted inxy-plane (lower) forQI1=10,QI2=70,QA1=170, andQA2=100. (b) Fluorescence micrograph of green and red tracer microbeads revealing the pathlines following a 2 s exposure. Position of the SP (indicated by the white arrow) can be deduced from the diverging path lines. In the lower micrograph, the SP moved from the centre towards the top-right and top-left apertures by∼97 and∼102 μm, respectively. (c) FEM modelization and (d) experimental results showing the asymmetric flow confinement and the gradient when the interface is straight (upper) and curved (lower) as a result of moving the SP. The gradient can be moved and adjusted rapidly as illustrated in theSupplementary Movie 4. Figure 6: Hydrodynamic positioning of the SP. The SP and the gradient floating between the streams were tuned by independently adjusting the flow rate of each pole of the MQ. ( a ) Streamlines of the flow showing the SP at the centre (upper) of the MQ for Q I1 = Q I2 =10 nl s −1 and Q A1 =Q A2 =100 nl s −1 , and shifted in xy -plane (lower) for Q I1 =10, Q I2 =70, Q A1 =170, and Q A2 =100. ( b ) Fluorescence micrograph of green and red tracer microbeads revealing the pathlines following a 2 s exposure. Position of the SP (indicated by the white arrow) can be deduced from the diverging path lines. In the lower micrograph, the SP moved from the centre towards the top-right and top-left apertures by ∼ 97 and ∼ 102 μm, respectively. ( c ) FEM modelization and ( d ) experimental results showing the asymmetric flow confinement and the gradient when the interface is straight (upper) and curved (lower) as a result of moving the SP. The gradient can be moved and adjusted rapidly as illustrated in the Supplementary Movie 4 . Full size image Alternatively, for scanning larger areas and reach positions outside the MQ's central area, the gradient at a point may also be changed by displacing the substrate relative to the MFP, either by moving the bottom substrate that is clamped to the motorized xy -stage of the microscope, or by manually moving the MFP using the micrometer screws of the probe holder ( Fig. 2c ) [21] . The MQ field lines and the concentration gradient are temporarily perturbed while the MFP moves relative to the substrate proportionally to the speed of displacement. For example, a speed of 300 μm s −1 lead to a small but visible disturbance of the gradient ( Supplementary Movie 5 ). The results indicate that the gradient re-equilibrated within few seconds after stopping the movement. Faster movements are possible but at the expense of greater disturbance of the gradient. Supplementary Movie 6 shows the gradient while moving the substrate at speed of 7 mm s −1 , and Supplementary Movie 7 shows the gradient while the MFP is being manually displaced. Using these two approaches, different areas of the substrates can be exposed to the gradient one after the other. We have presented an experimental demonstration of fluidic quadrupoles and found excellent agreement between theoretical prediction and experimental results, thus lending support to the general analytical framework developed to describe multipolar flow. Using the Hele–Shaw formalism, we established a close analogy between MQs, electrical quadrupoles, and vortex sheets in fluid dynamics. Our analysis was extended to include phenomena that were not studied before and the governing equations for a Hele–Shaw geometry derived for flow confinement and for the convection–diffusion of solutes at the SP. In analogy to electrical poles, and as was developed theoretically [11] , [16] , the number of poles may be further expanded and inspire combined theoretical and experimental studies of convection–diffusion phenomena with multiple poles and multiple chemicals. We demonstrated a first application of MQs as concentration gradient generators. The gradient is generated around the SP that experiences no flow and no shear stresses similar to stationary source-sink gradients [22] , [23] , while being continuously fed by the streams of the MQ and thus formed within seconds and could be rapidly adjusted, akin to microfluidic gradients with active flow [24] , [25] , [26] , [27] . Several approaches for forming gradients using hybrid approaches combining flow and no-flow zones have been proposed, but required porous elements [28] , [29] or nanochannels [30] , [31] . Gradients in open chambers have also been proposed [32] , [33] to allow user access (that is, pipetting) to the cell culture. These devices provide low shear stress cultures, while allowing to adjust the concentration gradients. However, these devices entail either closed chambers, or complicated fabrication processes, or both, and the time to adjust the gradient was typically longer than with the MQ. Another recent technique [34] used a laser beam to open and close pores in an integrated impermeable membrane to expose the cell culture to reagents selectively; however, this device involves closed cell culture chamber and a sophisticated experimental setup. The floating gradients formed within the MQ are remarkable because of a series of individual characteristics, and owing to the properties and possibilities that arise by the combination of these characteristics. They include, being open and brought down onto the target areas, the combination of active flow and shear-free zone obtained using hydrodynamic effects alone and without need for nanochannels or membranes, the possibility to rapidly adjust and move the gradient hydrodynamically within a few seconds, while also allowing to move it physically by displacing the MFP, and, finally, the possibility of repeated use of the device for many different experiments. This setup should be well suited for applications in cell biology such as studying cellular migrations [26] , [35] and neuronal navigation [36] , [37] , or stem cell differentiation [38] , because chemical cues can be applied and modulated rapidly to individual cells at the SP with minimal shear stress. It will be interesting to find out whether these properties can be exploited and the MFP–MQ used to study the response of neurons and stem cells to gradients; indeed neurons and stem cells are particularly difficult to culture and maintain inside closed channels for long periods [39] , [40] , and that have been shown to be very sensitive to shear stress [41] . Furthermore, the MQ and floating gradients could be used to study large samples that are hard to cultivate inside closed channels, such as embryos or tissue slices [42] . Finally, it may be useful for surface patterning by positioning and scanning the MFP atop surfaces [9] , [43] , [44] . The MFP fabrication and operation The MFP comprises a square Si chip (3 mm in width) with 4 etched holes of 360 μm diameter, and a PDMS interface chip with holes for receiving the capillaries of 360 and 250 μm outer and inner diameters, respectively, that connect it to the injection and aspiration syringe pumps (Nemesys) ( Fig. 2a ). The Si chips were fabricated in 200 μm thick, double-side-polished silicon wafers (Silicon Quest), using photolithography and deep-reactive-ion etching. Etching masks were formed on silicon wafers by using standard photolithography and S1813 photoresist (Shipley) to pattern a 2 μm thick thermal SiO 2 layer. The openings were made by deep reactive ion etching (DRIE, ASE etcher, Surface Technology Systems). The PDMS interface block was fabricated by casting poly(dimethylsiloxane) PDMS (Sylgard 184Dow Corning) into a home-made micromold composed of two structured steel plates, a polished steel plate with vias (access holes) forming the bottom, and four capillaries (each inserted into one of the four vias in the polished steel plate) serving as place holders for the fluidic connection holes. The PDMS was cured in an oven at 60 °C for at least 3 h (usually over night). The PDMS block was bonded to the Si chip by activating both parts in air plasma (Plasmaline 415 Plasma Asher, Tegal Corporation), at 0.2 mbar for 45 s at 75 W, and joining the two together using a home-made mechanical alignment aid and placed in an oven at 90 °C for 20 min. Operation of this MFP is similar to the use of the original MFP [9] , [21] , [44] , except that four independent syringe pumps are required to control the flow rate of each aperture independently. Briefly, the MFP was secured inside the clamping rode ( Fig. 2b ) and mounted on the xyz micropositioner (7600-XYZL, Siskiyou), what we call the probe holder. Using the probe holder, the MFP was positioned parallel to the transparent substrate (glass slide) atop an inverted microscope (TE2000, Nikon) so as to form a microscopic gap while immersed under the surrounding medium ( Fig. 2c ). Glass capillaries (Polymicro Tech) connect the MFP apertures to glass syringes (Hamilton) that are operated using a computer-controlled syringe pumps (Nemesys Cetoni). Numerical simulations The three-dimensional simulations were carried out using the commercially available finite element simulation software Comsol Multiphysics 3.5 (Comsol) and run on an eight-core, 64-bit computer (Xeon, Dell) with 26 GB of RAM. The MFP geometry was modelled with the same shape and dimensions as the microfabricated MFP used in the experiments. Simulations coupled the solution of Navier–Stokes equation and convection–diffusion equation. Sample solutions were assumed to be water (incompressible Newtonian fluid with a density of 998.2 kg m −3 , and a dynamic viscosity of 0.001 N·s m −2 ), and the diffusion coefficient of the solute was 500 μm 2 s −1 , which corresponds to the diffusion constant of fluorescein in water. The simulations were run under steady-state conditions and assumed no-slip boundary conditions on the substrate and the MFP surface, with the flow boundary conditions at the MQ's perimeter sides set as open boundaries (equal to atmospheric pressure). As boundary conditions for the mass transfer equation, the MFP surface and substrate were defined as an insulating boundary, and a zero inward flux was set at the perimeter of the MQ model. The experimental values were used for injection and aspiration flow rates. The concentration of the solute at the source injection aperture was arbitrarily set to 1 mol m −3 , 0 at the other injection aperture, and convective flux was set for both aspiration apertures. Image acquisition and analysis Images were recorded using a cooled CCD camera (Photometrics CoolSNAP HQ2) connected to the microscope. Black-and-white images were analysed and coloured using the software ImageJ 1.42 (National Institutes of Health Maryland). Images of green and red beads pathlines were joined together digitally using the freeware software GIMP 2.6.7 (Free Software Foundation). Videos were recorded using a digital consumer camcorder camera (HDR-SR7, Sony Electronics) connected to the microscope through a C-mount adaptor. The gradient lengths shown in Figure 5g were defined as the distance between 90 percent and 10 percent of the maximum fluorescence intensity signal, as shown in Supplementary Figure S5 . Chemicals and experimental procedures Fluorescein sodium salt (C 20 H 10 Na 2 O 5 ) was purchased from Sigma-Aldrich, and fluorescein solutions were prepared by dissolving 0.03 g of the salt with 100 ml of distilled water. Red and yellow-green carboxylate-modified fluorescent microspheres (fluosphere, 2 μm diameters) were purchased from Invitrogen. The solutions used in experiments were prepared by diluting 0.1 ml of the beads solution with 13 ml of distilled water. How to cite this article: Qasaimeh, M. A. et al . Microfluidic quadrupole and floating concentration gradient. Nat. Commun. 2:464 doi: 10.1038/ncomms1471 (2011).